A solution to the collective action problem in between-group conflict with within-group inequality Conflict with conspecifics from neighbouring groups over territory, mating opportunities and other resources is observed in many social organisms, including humans. Here we investigate the evolutionary origins of social instincts, as shaped by selection resulting from between-group conflict in the presence of a collective action problem. We focus on the effects of the differences between individuals on the evolutionary dynamics. Our theoretical models predict that high-rank individuals, who are able to usurp a disproportional share of resources in within-group interactions, will act seemingly altruistically in between-group conflict, expending more effort and often having lower reproductive success than their low-rank group-mates. Similar behaviour is expected for individuals with higher motivation, higher strengths or lower costs, or for individuals in a leadership position. Our theory also provides an evolutionary foundation for classical equity theory, and it has implications for the origin of coercive leadership and for reproductive skew theory. Social organisms living in stable groups often engage in aggressive interactions with conspecifics from neighbouring groups over territory, mating opportunities and other resources. The outcome of these interactions can significantly affect both individual fitness and group survival. Examples include border patrols in chimpanzees [1] , [2] , raiding parties in spider monkeys [3] , clan wars in hyenas [4] and between-group fights in lions [5] , free-ranging dogs [6] , meerkats [7] , Capuchin monkeys [8] , blue monkeys [9] , black howler monkeys [10] and ring-tail lemurs [11] . As in other collective activities that lead to the production of a public good, aggressive between-group interactions result in a collective action problem: if a group member benefits from the action of group-mates and individual effort is costly, then there is an incentive to ‘free ride’, that is, to reduce one’s effort or to withdraw it completely. However, if individuals follow this logic, the public good is not produced and all group members suffer. Overcoming the collective action problem is a major challenge facing social groups across a range of species, including humans [12] , [13] , [14] . Theoretical studies of cooperation have identified several possible solutions for reducing free-riding tendencies, such as altruism, relatedness, direct and indirect reciprocity, and punishment [15] , [16] . Although these mechanisms should in general also apply to cooperation in between-group conflict, theoretical and empirical work is limited in scope [17] . Here we investigate the collective action problem in between-group conflict within an evolutionary context. In particular, we study the effect of within-group inequality on provision of the public good, that is, differences between group-mates in dominance rank, status, motivation, valuation of the reward, costs paid and strength. We identify a mechanism that can overcome the collective action problem in groups of unrelated individuals without recourse to altruism, reciprocity or punishment. Our focus is on the evolution of social instincts. As first argued by Darwin in On the Origins of Species , social instincts—that is, genetically based propensities that govern the behaviour of individuals in social interactions—have evolved by natural and sexual selection. In modern perspective, these instinctive social behaviours are plastic, resulting from the interaction of the genotype with the social environment (including the behaviour of social partners) [18] . By focusing on the origin of social instincts, the framework we develop here aims to place the debate [19] on between-group conflict in human evolution within a broad cross-specific perspective. A crucial evolutionary question, discussed already by Darwin in The Descent of Man , is how important between-group conflict was in shaping the human behavioural repertoire. Existing theoretical work suggests that relatively modest levels of mortality in between-group conflict could have sufficiently large evolutionary effects, driving the emergence of characteristic human abilities, biases and preferences (for example, cooperation, altruism, belligerence, parochialism and ethnocentrism), as well as social and cultural norms and institutions [16] , [20] , [21] , [22] , [23] , [24] . Like Darwin’s account, these theoretical approaches rely on factors that are exclusive to our species, such as cultural transmission aided by language, culturally enforced sharing norms or group decisions and particular within- and between-group interaction patterns (for example, cultural group selection) [16] , [22] . Given that our approach does not rely on these factors, our insights may apply to any species with between-group conflict. This body of theoretical work is informed by inferences drawn from comparison with the social systems of other primate species, or from archaeological and ethnographic data [16] , [25] , [26] , [27] , [28] , [29] , [30] . Many of these inferences are contentious [19] . For example, the ethnographic data typically pertain to present-day mobile forager groups, which are characterized by an egalitarian social structure [31] . However, it is not clear to what extent this social system is a good ‘model’ for early human groups. Other types of small-scale societies may also provide clues to early human social systems, but they have been largely neglected in the literature on the evolution of cooperation. This includes semisedentary and sedentary forager groups with varying degrees of hierarchy and other types of inequality. Our work may provide insights into the dynamics of these groups and guide discussions of human cooperation towards a broader conceptual framework. Our models are grounded in contest theory, an approach used widely in economics [32] . We extend in several important directions existing work on the evolution of cooperation in the context of between-group conflict. First, rather than allowing for only two discrete strategies (for example, cooperate and defect), we use a more general and realistic framework in which individual efforts and costs are treated as continuous variables; this is also more in line with experimental economic games, where subjects can typically vary their contributions continuously. Second, existing models of between-group conflict use standard public goods games, where individual benefit is a linear function of the number of contributors (or of their total effort). However, it is now recognized that this assumption can lead to misleading conclusions [32] , [33] . In our approach, benefits are specified by a nonlinear function explicitly capturing the efforts of both focal and competing groups. Third, existing approaches postulate a completely egalitarian division of spoils and disregard any differences between individuals except for the strategy they use. In contrast, as noted above we explicitly aim to capture the effects of differences between individuals on their strategies and the fitness consequences of their actions (for example, differences with respect to their dominance rank, status, motivation, valuation of the reward, costs paid and strength). Finally, compared with related work in the economics literature [32] , [34] , our approach adds biological realism by focusing on evolution by small mutations, by explicitly allowing for group extinction and multiplication and by investigating the effects of migration and genetic relatedness. Here we study a series of mathematical models describing competition between groups comprising heterogenous individuals. Our models show that within-group inequality leads dominant individuals (or those with higher strengths or lower costs) to contribute the effort required to produce the public good (that is, to succeed in between-group competition) while the rest of the group free rides [12] . This is because they can ‘afford’ higher costs of contribution, owing to their larger shares of the public good. Their behaviour is seemingly altruistic, in the sense that they contribute more effort than their group-mates and often have lower fitness as a result. Their contribution is driven by competition with their counterparts in other groups rather than with their own group-mates. This mechanism can overcome the collective action problem in groups of unrelated individuals without resorting to altruism, reciprocity or punishment. Basic model We consider a population of individuals living in a large number of groups G of constant size n . The groups engage in competition for resources, which affects their survival and multiplication as well as the reproduction of members of surviving groups. Groups can be egalitarian, so that each individual gets an equal share of the resources that the group obtains, or hierarchical, so that each individual’s share depends on its dominance rank. Each group faces a collective action problem. The amount of resources obtained by each group depends on the total effort of its members towards the group success; at the same time, individuals pay fitness costs that increase with their efforts. Each individual’s effort is controlled genetically and is modelled as a non-negative continuous variable. In the case of hierarchical groups, individual efforts are conditioned on the dominance rank, which is assigned to group members randomly at each generation (for example, based on their strength). There is no coercion. We allow for mutation, recombination, migration and genetic relatedness between individuals. To introduce our approach and results, we start with a simple model. Let P j be a share of the resources obtained by group j in competition with other groups, and x ij the effort of individual i in group j towards the group’s success ( i =1,…, n ; j =1,…, G ). We specify the total group effort as where the sum is taken over all group members, and define the group success probability P j as where the sum is taken over all groups [32] , [35] . We assume that the groups survive to leave offspring to the next generation with probabilities equal to P j . For members of such groups, we define individual fertility as where f 0 is a constant baseline fertility (which can be set to 1 without loss of generality), B is the total (normalized) resource contested by the groups, c is the cost parameter and v i is the share of the group’s reward allocated to individual i . We treat valuations v i as constants dependent on the within-group dominance rank ( v 1 ≥ v 2 ≥…≥ v n ; ∑ v i =1). The groups that do not survive are replaced by the offspring of surviving groups. Generations are discrete and non-overlapping. Specifically, we assume that each group in the current generation descends from a group in the previous generation chosen randomly and independently with probabilities P j . Individuals in each group descend from individuals in their parental group independently with probabilities , where is the average fertility in group j (=Σ i f ij / n ). Under these assumptions, the fitness of individual i from group j is In what follows it will be convenient to use parameter b = B /( nG ), which is the expected benefit per individual in an egalitarian group if all individuals in the population are identical. Below we describe our key findings. A technical explanation and derivations of our results are given in the Methods. Egalitarian groups Consider first the case when groups are egalitarian so that v i =1/ n for all i . Then, the population is predicted to evolve to an equilibrium at which the total group effort is while each individual effort is = X */ n . As expected, both individual and group efforts increase with benefit b and decrease with cost c . Increasing the group size n (while keeping b constant) does not change the total group effort, but it decreases the individual effort as a result of increasing free riding. If the benefit per individual b decreases with group size n , then the total group effort will decrease with increasing n . These results assume that the groups are formed uniformly at random each generation, implying that group members are no more genetically related to one another than they are to members of other groups. The evolution of cooperation in a public goods game as studied here is driven by the overlapping interests of group-mates [36] and does not require genetic relatedness (or reciprocity, coercion or punishment) [33] , [37] . Genetic relatedness does however increase cooperation [15] . In the model considered here, with average within-group relatedness r and no between-group relatedness, each individual effort increases by factor For example, let female offspring disperse randomly between groups while male offspring stay in the natal group (as in chimpanzees and, likely, in our ancestors [38] ). This will result in a ~30% increase in the individual and group efforts relative to the case of zero relatedness (assuming that n ≥5). Hierarchical groups The results outlined above assume a completely egalitarian division of the spoils. In hierarchical groups, the predicted collective action behaviour is strikingly different. With random group formation, only individuals with valuations v i higher than a certain threshold will make a non-zero effort, while low valuators will free ride contributing nothing. All ranks will contribute only if, for each i , Note that the threshold value v crit is close to 1/ n if the group size n and/or benefit b are large. If all ranks do contribute, then the total group effort X *=(1+ b )/ c , which is the same as in egalitarian groups. Ranks for which v i < v crit will contribute nothing. Counter-intuitively, the total group effort X * increases as the number of contributing ranks n e decreases. This happens because the remaining high-valuation contributors increase their efforts, effectively overcompensating for the lack of effort by the free-riding ranks. Individual effort x i * increases with valuation v i ; counter-intuitively, however, the individual fertility of contributing ranks decreases with valuation. That is, high-rank group members have lower fertility than their low-rank group-mates. This results from their increasing efforts and the correspondingly higher costs they pay, which negate the higher share of the reward that they claim. (For non-contributing ranks, fertility increases with valuation v i ). The above inequality is a necessary but not sufficient condition for rank i to contribute. (A recursive sufficient condition is given in the Methods). Because of this threshold effect, small differences in valuation can result in large differences in efforts and reproductive success. In the extreme case when only the highest valuator contributes effort, its share of group reproduction is the smallest in the group (and it is smaller than 1/ n ), in spite of this individual getting the highest share of the reward. 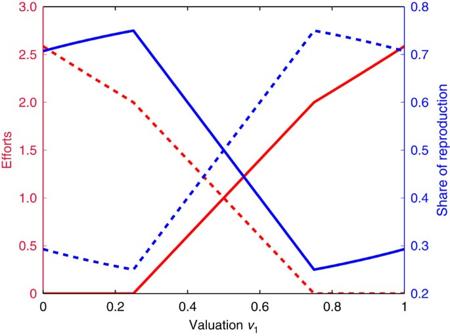Figure 1: Collective action in groups of sizen=2 with benefitb=1. Red lines show individual effortsxiand blue lines show the shares of reproductionfi/(f1+f2) for individuals 1 (solid lines) and 2 (broken lines). Both individuals contribute only if their valuations are larger than 0.25, otherwise the individual with the smaller valuation free rides. Figure 1 illustrates our results for the case of only two individuals per group ( n =2), which is a common set-up in reproductive skew theory [39] , [40] . Note that increasing the valuation increases fitness only if the individual free rides or if it is the only contributor. Otherwise, increasing the valuation decreases its share of reproduction. Figure 1: Collective action in groups of size n =2 with benefit b =1. Red lines show individual efforts x i and blue lines show the shares of reproduction f i /( f 1 + f 2 ) for individuals 1 (solid lines) and 2 (broken lines). Both individuals contribute only if their valuations are larger than 0.25, otherwise the individual with the smaller valuation free rides. Full size image Increasing the value of the resource b while keeping n fixed increases both individual efforts and the share of the effort contributed by rank-1 individuals. At the same time, this decreases their reproductive success because of increasing costs. Increasing the degree of inequality increases the group effort and can, counter-intuitively, increase the reproductive success of low-rank individuals. The key insight is that high-rank individuals behave seemingly altruistically: they contribute effort to the collective action at a cost, which reduces their fitness compared with their free-riding lower-rank group-mates. This behaviour is however not altruistic: they are maximizing their fitness by contributing, because they would not be better off by reducing their contribution or by not contributing. These individuals are essentially competing with high-rank individuals in the other groups, rather than with their own group-mates. Numerical simulations To confirm our conclusions using a more realistic description of the population structure, limited dispersal and the resulting genetic relatedness, we used individual-based simulations (see Methods). All individuals were haploid. The effort at each rank was controlled by an independent unlinked locus with a continuum of effects. Each group comprised n males and n females. Only males contributed to group competition and received benefits proportionally to their valuations. Females from surviving groups had equal reproductive success and each female produced two offspring. The fathers were chosen among the group males proportionally to their fertilities f i . The offspring sex was assigned randomly, but an equal sex ratio was enforced within each group. Female offspring dispersed randomly while male offspring stayed in the natal group. Numerical simulations show that, relative to the case of random group formation, genetic relatedness increases individual and group efforts and causes more low valuators to start contributing towards the group’s success. The overall effect is however not large because relatedness remains relatively low (see Supplementary Figs 1–6 ). Figures 2 , 3 , 4 illustrate our results using a model in which individual valuations are proportional to a power function of individual rank: v i ~( n +1− i ) δ . Here δ is a parameter measuring the degree of inequality: with δ =0, all valuations are equal to 1/ n , with δ =1 valuation v i is a linear function of individual rank i and with δ >1 it is a decreasing, concave-up function of rank. In simulations, we used five values of δ =0.25, 0.5, 1, 2, 4. 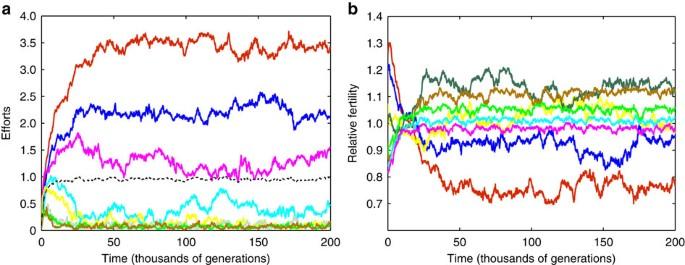Figure 2: Collective action in the basic model. Results over 200,000 generations for a particular run with group sizen=8 and within-group inequalityδ=2. The values are averages over individuals of rankiin all groups in the population. Colours describe different ranks, from rank 1 (red) to rank 8 (dark green). (a) Individual effortsxifor ranki; the average individual effort over all ranks is shown with the dashed line. (b) Relative fertilitiesfor individuals of ranki. Figure 2: Collective action in the basic model. Results over 200,000 generations for a particular run with group size n =8 and within-group inequality δ =2. The values are averages over individuals of rank i in all groups in the population. Colours describe different ranks, from rank 1 (red) to rank 8 (dark green). ( a ) Individual efforts x i for rank i ; the average individual effort over all ranks is shown with the dashed line. ( b ) Relative fertilities for individuals of rank i . 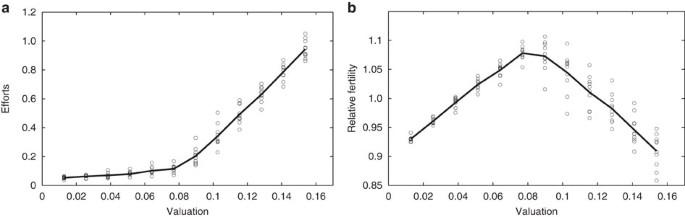Figure 3: Collective action in the basic model. Summary results of the last 20,000 generations for a particular set of 10 runs with group sizen=12 and within-group inequalityδ=1, as a function of individual valuationvi. For each run, the values are averages over individuals of rankiin all groups in the population. Values for individual runs are given by circles, the average over the 10 runs is given by a solid line. (a) Individual effortsxifor ranki. (b) Relative fertilitiesfor individuals of ranki. Full size image Figure 3: Collective action in the basic model. Summary results of the last 20,000 generations for a particular set of 10 runs with group size n =12 and within-group inequality δ =1, as a function of individual valuation v i . For each run, the values are averages over individuals of rank i in all groups in the population. Values for individual runs are given by circles, the average over the 10 runs is given by a solid line. ( a ) Individual efforts x i for rank i . ( b ) Relative fertilities for individuals of rank i . 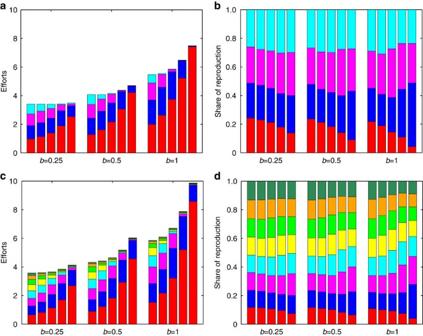Figure 4: Collective action in the basic model. Summary results over all runs for one set of parameters, with group sizen=4 (a,b) andn=8 (c,d) and costc=0.5. For each set of runs, the values are averages over individuals of rankiin all groups in the population. Colours show the relevant amounts for individuals of different ranks, from the rank-1 individual at the bottom (red) to the rank-nindividual at the top. Each set of bars corresponds to a specific value of benefitb. Each bar within a set corresponds to a specific value of within-group inequalityδ, from the smallest on the left (δ=0.25; low inequality) to the largest on the right (δ=4; high inequality). (a) Individual effortsxifor rankiwith group sizen=4; the height of the bar is the total group effortX*. (b) Share of reproduction for individuals of rankiwith group sizen=4. (c) Individual effortsxifor rankiwith group sizen=8; the height of the bar is the total group effortX*. (d) Share of reproduction for individuals of rankiwith group sizen=8. Full size image Figure 4: Collective action in the basic model. Summary results over all runs for one set of parameters, with group size n =4 ( a , b ) and n =8 ( c , d ) and cost c =0.5. For each set of runs, the values are averages over individuals of rank i in all groups in the population. Colours show the relevant amounts for individuals of different ranks, from the rank-1 individual at the bottom (red) to the rank- n individual at the top. Each set of bars corresponds to a specific value of benefit b . Each bar within a set corresponds to a specific value of within-group inequality δ , from the smallest on the left ( δ =0.25; low inequality) to the largest on the right ( δ =4; high inequality). ( a ) Individual efforts x i for rank i with group size n =4; the height of the bar is the total group effort X *. ( b ) Share of reproduction for individuals of rank i with group size n =4. ( c ) Individual efforts x i for rank i with group size n =8; the height of the bar is the total group effort X *. ( d ) Share of reproduction for individuals of rank i with group size n =8. Full size image Figure 2 illustrates the dynamics of individual efforts and fertilities with n =8. In this case, only the top three ranks make substantial contributions. (Note that because of mutation individual contributions always remain positive). Figure 3 shows the average efforts and fertilities for different ranks with n =12. The ranks with the lowest valuations contribute almost nothing and their fertilities increase with valuation. The contributions of the high valuators increases linearly with v i but their fertilities decrease linearly with v i . Figure 4 is a summary graph showing that as within-group inequality increases (measured by δ ), the individual efforts of high valuators increase while their shares of reproduction decrease. They also show that the total group effort grows with within-group inequality and benefit b . Generalizations To check the robustness of our conclusions, we have also studied two modifications of the basic model. In the first version, the probability of group success was specified as where β is a positive parameter measuring the ‘decisiveness’ of the group strength: β >1 implies that stronger groups will get disproportionately large shares of the reward [32] . Increasing β increases both the individual and group efforts (as expected), but it results in no other qualitative differences ( Fig. 5 ). 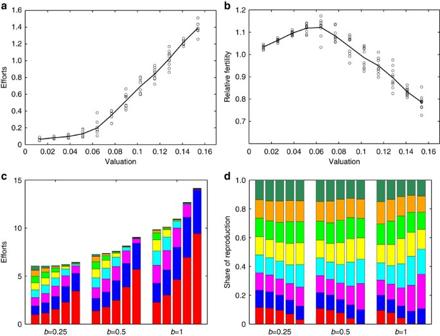Figure 5: Collective action in the modified model with decisivenessβ=2. Group sizen=8 and costc=0.5. (a,b) Summary results of the last 20,000 generations for a particular set of 10 runs with within-group inequalityδ=1, as a function of individual valuationvi. For each set of runs, the values are averages over individuals of rankiin all groups in the population. Values for individual runs are given by circles, the average over the 10 runs is given by a solid line. (a) Individual effortsxifor ranki. (b) Relative fertilitiesfor individuals of ranki. (c,d) Summary results over all runs for one set of parameters. For each run, the values are averages over individuals of rankiin all groups in the population. Colours show the relevant amounts for individuals of different ranks, from the rank-1 individual at the bottom (red) to the rank-8 individual at the top (dark green). Each set of bars corresponds to a specific value of benefitb. Each bar within a set corresponds to a specific value of within-group inequalityδ, from the smallest on the left (δ=0.25; low inequality) to the largest on the right (δ=4; high inequality). (c) Individual effortsxifor ranki; the height of the bar is the total group effortX*. (d) Share of reproduction for individuals of ranki. Figure 5: Collective action in the modified model with decisiveness β =2. Group size n =8 and cost c =0.5. ( a , b ) Summary results of the last 20,000 generations for a particular set of 10 runs with within-group inequality δ =1, as a function of individual valuation v i . For each set of runs, the values are averages over individuals of rank i in all groups in the population. Values for individual runs are given by circles, the average over the 10 runs is given by a solid line. ( a ) Individual efforts x i for rank i . ( b ) Relative fertilities for individuals of rank i . ( c , d ) Summary results over all runs for one set of parameters. For each run, the values are averages over individuals of rank i in all groups in the population. Colours show the relevant amounts for individuals of different ranks, from the rank-1 individual at the bottom (red) to the rank-8 individual at the top (dark green). Each set of bars corresponds to a specific value of benefit b . Each bar within a set corresponds to a specific value of within-group inequality δ , from the smallest on the left ( δ =0.25; low inequality) to the largest on the right ( δ =4; high inequality). ( c ) Individual efforts x i for rank i ; the height of the bar is the total group effort X *. ( d ) Share of reproduction for individuals of rank i . Full size image In another modification, we assumed that group-mates share the reward equally ( v i =1/ n ) but differ with respect to the cost coefficient c i . This may be the case if some individuals are stronger than others, so that the same amount of effort can be less costly for them in fitness terms. In our simulations, we used costs c i that increased linearly with rank i . Specifically, we used n equally spaced values of c i from (1− d )/2 to (1+ d )/2 with five different values of d : 0.05 (small differences in costs), 0.1, 0.2, 0.4, 0.8 (large differences in costs). Our major conclusions remain qualitatively valid, with low-cost individuals playing the role of high-valuation group members in the basic model ( Fig. 6 ). 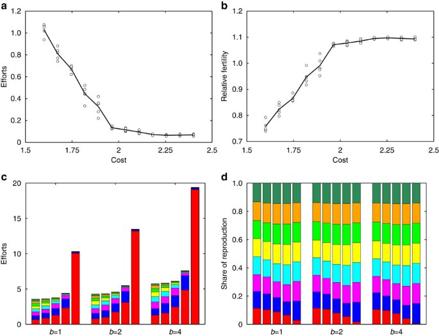Figure 6: Collective action in the modified model with individual costsciincreasing linearly with ranki. Group sizen=8 and egalitarian division of spoils (that is, the individual shares of the reward arevi=1/nfor alli). (a,b) Summary results of the last 20,000 generations for a particular set of five runs with within-group inequalityd=0.2, as a function of individual costci. For each run, the values are averages over individuals of rankiin all groups in the population. Values for individual runs are given by circles, the average over the five runs is given by a solid line. (a) Individual effortsxifor ranki. (b) Relative fertilitiesfor individuals of ranki. (c,d) Summary results over all runs for one set of parameters. For each set of runs, the values are averages over individuals of rankiin all groups in the population. Colours show the relevant amounts for individuals of different ranks, from the rank-1 individual at the bottom (red) to the rank-8 individual at the top (dark green). Each set of bars corresponds to a specific value of benefitb. Each bar within a set corresponds to a specific value of parameterdcontrolling differences in costs, from the smallest on the left (d=0.05; small difference in costs) to the largest on the right (d=0.8; high difference in costs). We usednequally spaced values of individual costscifromc× (1−d)/2 toc× (1+d)/2. (c) Individual effortsxifor ranki; the height of the bar is the total group effortX*. (d) Share of reproduction for individuals of ranki. Note that the model with differences in costs is mathematically equivalent to a model with a constant cost c but with differences in fighting abilities s i and the total group effort defined as Figure 6: Collective action in the modified model with individual costs c i increasing linearly with rank i . Group size n =8 and egalitarian division of spoils (that is, the individual shares of the reward are v i =1/ n for all i ). ( a , b ) Summary results of the last 20,000 generations for a particular set of five runs with within-group inequality d =0.2, as a function of individual cost c i . For each run, the values are averages over individuals of rank i in all groups in the population. Values for individual runs are given by circles, the average over the five runs is given by a solid line. ( a ) Individual efforts x i for rank i . ( b ) Relative fertilities for individuals of rank i . ( c , d ) Summary results over all runs for one set of parameters. For each set of runs, the values are averages over individuals of rank i in all groups in the population. Colours show the relevant amounts for individuals of different ranks, from the rank-1 individual at the bottom (red) to the rank-8 individual at the top (dark green). Each set of bars corresponds to a specific value of benefit b . Each bar within a set corresponds to a specific value of parameter d controlling differences in costs, from the smallest on the left ( d =0.05; small difference in costs) to the largest on the right ( d =0.8; high difference in costs). We used n equally spaced values of individual costs c i from c × (1− d )/2 to c × (1+ d )/2. ( c ) Individual efforts x i for rank i ; the height of the bar is the total group effort X *. ( d ) Share of reproduction for individuals of rank i . Full size image In this model, individuals with larger fighting abilities s i will, ceteris paribus , contribute more to X . Therefore, our conclusions are applicable to the case of within-group variation in strengths. That is, lower-cost or higher-strength individuals are predicted to contribute more effort than their group-mates, and they can have lower reproductive success as a result. We have studied the collective action problem in between-group conflict within an evolutionary context, focusing on the effect of within-group inequality in dominance rank, status, motivation, valuation of the reward, costs paid and strength. We have shown that inequality in rank can lead dominant individuals to act seemingly altruistically towards their group-mates by contributing the effort required to succeed in between-group competition while others free ride. As a result, these individuals have reduced reproductive success compared with their free-riding subordinate group-mates. Analogous reasoning applies when individuals differ in the costs incurred from contributing to the public good or when they differ in strength: lower-cost or higher-strength individuals contribute more effort to the public good, and they have reduced reproductive success compared with their free-riding group-mates as a result. This behaviour may seem altruistic but actually it is not. In the case of hierarchical groups, for example, dominant individuals maximize their fitness by contributing; given the subordinates’ lack of contribution, dominants will not be better off by reducing their contribution or by withholding it completely. Thus, the non-contributors are indeed free riding, but the contributors are not altruistic; paradoxically, they are acting in their own interest by contributing to the public good. What is driving their contribution is that they are essentially competing with their counterparts in other groups rather than with their own group-mates. The outcome of seemingly altruistic behaviour by dominant individuals (or those with lower costs or higher strength) is consistent with Olson’s controversial conclusion that individuals who obtain the greatest share of a public good bear a disproportionate share of the costs, leading to ‘ a systematic tendency for ‘exploitation’ of the great by the small !’ [12, (p. 29)]. Olson’s insight relates to the phenomenon of collective action within a single group. Here we have shown that this effect can be even more extreme when the driving force of collective action is between-group conflict coupled with within-group inequality. In this case, groups of unrelated individuals can ‘solve’ the collective action problem without resorting to altruism, reciprocity or punishment. Note that we assumed that individual efforts are only limited by the requirement of non-negative fertility ( cx i <1+ bnv i ). However, if there is a smaller upper limit on x i (for example, due to physiological, energetic or time constraints), then a single individual (or a small group) may not be able to contribute the optimum effort predicted by our theory. In this case, we expect that the number of contributors will increase [34] relative to our predictions. Our work has connections with several other classes of models and results in behavioural biology; here we outline some of the similarities, differences and their implications. The mechanism for the evolution of seemingly altruistic behaviour we identify is analogous to the emergence of ‘altruistic’ soma in multicellular organisms [41] , but without the need for genetic relatedness. Our results show that within-group genetic relatedness increases the ‘altruistic’ effort of dominant individuals but is not required for the mechanism to operate. The system state with heterogenous groups in which only some individuals make an effort while the rest free ride is somewhat similar to polymorphic states observed in producer–scrounger models [42] , [43] . In these models, some individuals pay fitness costs to discover resource items, while the rest avoid these costs by using the resources discovered by others. The major difference is that while in classical producer–scrounger models the two strategies have equal fitness at equilibrium, in between-group conflict ‘producers’ (that is, contributors) have lower fitness than their free-riding group-mates. Our insights on hierarchically structured groups bear on work on reproductive skew, the unequal partitioning of reproduction within a group [39] , [40] . Models in reproductive skew theory focus on the evolution of investment in within-group competition (for example, by dominant versus subordinates), given its negative effect on between-group competition and given genetic relatedness between group members. In contrast, we assume that the within-group division of benefits is set by factors endogenous to the model (for example, based on rank), and we study the evolution of costly investment in between-group competition. In our models, genetic relatedness is of secondary importance. Most of the modelling work on reproductive skew involves groups with two reproductive classes and linear production functions. Our results and techniques for groups of arbitrary size and nonlinear production functions can be used to obtain additional insights into the evolution of reproductive skew. For example, a key question in this area is why some individuals (for example, subordinates) ‘stick around’ in stable groups when other individuals (for example, dominants) monopolize a disproportionate share of reproductive opportunities [39] , [40] . Qualitatively, one insight from our work is that, in between-group conflict scenarios, subordinates can reap the benefits of collective action without bearing any costs, which are borne instead by dominant individuals. This may provide an incentive for subordinates to stay in the group. Thus, while in reproductive skew theory subordinate individuals are commonly viewed as making ‘the best of a bad job’, in our models they are in fact better off than dominant individuals. In hierarchical groups, dominant individuals are able to bully their group-mates, typically usurping a disproportional share of material resources and mating opportunities. Reducing the negative effects of dominant bullies on their group-mates requires the formation of coalitions between subordinates [31] , [44] , [45] , [46] . Our theory predicts that, at the same time, dominant bullies may act ‘altruistically’ towards their group-mates in between-group conflict situations. As we saw above, this is because, once a within-group hierarchy is established, alpha-individuals effectively compete against alpha-individuals in other groups rather than against their own group-mates; the competition can drive the within-group fitness of alpha-individuals to very low values. Note that this only applies to public goods contested by groups: if a group survives the between-group conflict, then there are other resources that dominant individuals can seize from their group-mates in within-group interactions. Therefore, high-rank individuals are not necessarily worse off in terms of overall fitness. A final connection is with the growing literature on the evolution of leadership and followership and on the psychological mechanisms underlying these traits in humans. One of the roles ascribed to leaders in this literature is punishment of defectors in collective action [47] , [48] or punishment of individuals who disrupt group cohesion [49] . Our models do not allow for punishment. However, our results suggest that, were this included, dominant individuals in hierarchical groups may evolve the tendency to punish low-rank free riders to increase their effort in collective action. This expectation is reinforced by the results of experimental economic games showing that between-group competition enhances punishment of free riders [50] ; they also show that, when individuals are heterogenous with respect to the costs of administering punishment, the tacit expectation is that punishment will be carried out by the group member with the smallest cost [51] . An open question is how exactly individuals will partition their effort between punishing their group-mates and contributing directly to between-group competition. Overall, our models predict higher effort for high-rank individuals towards collective action in between-group competition. This is consistent with empirical observations across a range of species, including humans. In chimpanzees, high-rank males travel further into the periphery during border patrols [2] and males with higher mating success are more likely to engage in this activity [1] , which is energetically costly [52] . In ring-tail lemurs [11] and blue monkeys [9] , high-rank females participate more in the defence of communal feeding territories than low-rank females; note that in both species, males disperse from the natal group, that is, the dispersal pattern is reversed compared with the scenario captured by our simulation set-up. In meerkats, dominant males respond more strongly to intruder scent marks [53] . High-rank chacma baboon males are more likely than low-rank males to join inter-group loud call displays [17] . In some human groups, the most aggressive warriors have lower reproductive success than other men, as documented for the horticulturalist/forager Waorani of Ecuador [54] . Our results are also relevant for explaining the propensity to sacrifice (that is, to expend relatively more effort) of individuals in leadership positions in warfare and other between-group competition scenarios. For example, the highest mortality in the US Army in the Iraq War was among First and Second Lieutenants, who typically lead combat patrols [55] . Note that we predict higher efforts and costs not only for individuals who actually hold or have been assigned high rank or status, but also for ‘potential alphas’ who have higher valuation of the prize, lower costs or higher strength. Finally, our work suggests that bullish and ‘unethical’ behaviour by high-rank individuals towards their group-mates [56] will be accompanied by their higher contributions towards between-group competition. Although experimental studies of public good games with between-group competition [57] , [58] , [59] typically do not allow for within-group variation in valuation, the data available for humans do show that more competitive, individualistic players contribute more to public goods with group competition [60] and that individuals of high status contribute more towards group goals [61] . We conclude our discussion by outlining some implications that apply specifically to human behaviour. One set of implications relates to the emergence of an evolved psychology for egalitarian tendencies in hierarchical groups [46] . This process is linked to the intentional eradication of dominant bullies (and their genes) by their group-mates, as in the ‘reverse dominance hierarchies’ of present-day mobile forager groups [31] , [44] . In related studies, Bowles and co-authors have argued that genes for altruism can proliferate relatively easily in the presence of culturally enforced leveling mechanisms, such as meat sharing. This would have resulted in greater efficiency of egalitarian groups in between-group conflict, leading to the emergence of an egalitarian social structure via cultural group selection [62] , [63] . Our work offers a different perspective. First, our results show that high-rank bullies make key contributions in between-group conflict and that ‘despots’ can dialectically become ‘altruists’. Such individuals may have played an important role in human social evolution and genes for such behaviour may have been maintained in the population by selection. Second, in our models the total group effort typically increases with the degree of inequality. (If all group members contribute, then the total group effort does not depend on the degree of inequality). This implies that hierarchical groups will expend more effort in between-group conflict and are thus likely to outcompete more egalitarian groups. Overall, our theory suggests that humans may have stronger innate preferences for an egalitarian social structure in the absence of between-group conflict [46] and for a hierarchical social structure in its presence. Egalitarian groups are subject to stronger overall free riding and as a result they may allocate less effort to between-group conflict. More broadly, our work adds a new mechanism to those commonly invoked to explain the evolution of cooperation in humans. This mechanism does not rely on factors that are exclusive to our species (for example, cultural transmission aided by language) or traits characteristic of a particular type of human social system (for example, the leveling mechanisms attributed to mobile forager groups). Our work thus extends the range of information that can be brought to bear on questions about human social evolution. A final implication of our work that applies specifically to human behaviour relates to the origin of fairness norms. Social instincts that evolved under ancestral conditions of between-group conflict may also affect preferences and biases exhibited in peaceful collective activities, such as one’s day job. If people feel that they are fairly compensated, then they are generally happier at work and more motivated to continue contributing input at the same level. But what is the ‘fair’ compensation when individuals involved in a collective project are unequal in their roles and types of inputs? The answer provided by classical equity theory [64] , [65] is that employees seek to maintain equity between their input-to-output ratio and that of others. (The theory does recognize that the ‘input’ of workers includes many factors besides working hours, and that their ‘output’ includes many rewards besides money). Although equity theory has attracted a number of consistent criticisms, including the lack of evolutionary foundations [65] , it remains one of the more important and successful theories in the field of organizational behaviour. While the expectation of a positive relationship between output and input seems quite natural, why this relationship should be linear (as postulated in equity theory) rather than, say, quadratic is a priori unclear. In our models, evolution adjusts the efforts of contributing individuals so that they become linearly aligned with the individual shares of the reward emerging from the collective action ( Figs 3a and 5a ). Thus, our results provide a theoretical evolutionary foundation for a major assumption of classical equity theory. Clearly, in collective action as in other domains, human behaviour is greatly influenced by cultural institutions, societal norms, the possibility of punishment, preferences, emotions and so on [31] , [44] . Human history provides many examples of norms and institutions that reduce free riding in more egalitarian groups, making them efficient in competition. For instance, early eighteenth century pirates formed effective predatory groups and had a relatively ‘flat’ structure: the captain’s share of the booty was only twice as large as the share of an ordinary crew member [66] . In the context of business organizations, the advantages of hierarchical versus more egalitarian firms in competition with one another are currently hotly debated [67] , [68] . Hence, the theory outlined here, with its exclusive focus on the emergence of genetically controlled social instincts, is only part of the picture. However, we contend that this is an important part—one that helps us ground the evolution of human behaviour within a broad cross-specific perspective. Fitness In our models, the fitness of individual i from group j can be written as To study our models, we use the evolutionary invasion analysis (adaptive dynamics [69] ) approach, which focuses on the invasion fitness w ( y | x ), that is, the fitness of a rare mutant with trait y in a monomorphic population of individuals with trait x . We assume that the effort for each rank is specified genetically and that there is only a single segregating mutation across all the ranks at any one time. Egalitarian groups Assume that group members share the reward equally so that nv i =1 for each i . To evaluate the change in individual effort x per generation, one needs to calculate the selection gradient of the invasion function at y = x . To find the invasion fitness w ( y | x ), we need to set x ij = y , , f ij =1+ bGP j − cy , and in equation (10). In the limit of large G , the selection gradient at y = x is proportional to 1+ b − cnx . Then, one finds that at equilibrium Summing up the individual contributions, the total group effort X *=(1+ b )/ c and thus it does not depend on n . Let r 0 and r 1 be the probabilities that a randomly chosen group-mate of a mutant and a randomly chosen individual from a different group have the same mutation. Then, the equilibrium effort x * is increased by a factor Note that if female offspring disperse randomly between groups while male offspring stay in the natal group, the males within the group will be genetically related with average relatedness [70] . If the number of groups is large, r 1 will be very close to zero. Assume that the probability of success is . Then, One can show that with relatedness and decisiveness, the total group effort X * increases with the group size n (assuming r 1 << r 0 ). Hierarchical groups Assume that group members differ in their valuations v i and that each group is characterized by exactly the same set of v i values. To find the invasion fitness w ( y i | x i ) for the effort x i at rank i , we need to set x ij = y i , f ij =1+ bGP j nv i − cy i , , and in equation (10). Here X =∑ j x j and X − i = X − x i . Then, in the large G limit, the selection gradient at y = x for x i is proportional to This equation is linear in x i . It follows that effort x i at each rank i evolves either to a positive value or to zero. Assume first that the effort at each rank evolves to a positive value . Summing up equation (16) over all i with account that ∑ v i =1 and ∑ x i = X , one finds that X satisfies to a quadratic equation Therefore, at equilibrium (The other solution, X *= n (1+ b )/ c , results in zero average fertility and thus is not biologically relevant). That is, the total group effort does not depend on the group size or on the distribution of the valuations. The equilibrium individual efforts are This equilibrium is feasible (that is, all x i *>0) if for all i Note that increasing the value of the resource b or the group size n moves v crit closer to 1/ n , so that individuals with a valuation smaller than the average will not contribute but will free ride. Equation (19) shows that individual efforts increase with valuation v i . In contrast, individual reproductive success at equilibrium is and thus decreases with valuation. That is, the higher costs paid by high-rank individuals negate their larger shares of the reward. If not all group members make a positive effort, then the derivations become more complex. Let there be n e contributors and v be their total valuation ( v =∑ v i where the sum is over n e contributors). Then, summing up equation (16) over all contributors, at equilibrium their total effort X satisfies to a quadratic equation Of the two solutions of this quadratic, only the smallest one, X *, is relevant biologically (the other solution leads to negative fertilities). Note that cX *≤ n e + bn Σ v i < n (1+ b ). (The first inequality follows from the requirement that all f i values are non-negative: , which one then sums up over all contributing individuals). The individual efforts can be found from equation (16) by substituting X * into This equilibrium is biologically feasible (that is, all ), if Equation (23) shows that individual effort increases with valuation. However, within-group reproductive success and is decreasing with valuation v i because cX *≤ n ( b +1). By differentiating the expression for X *, one can show that X * always increases with v and generally decreases with n e . (The latter requires that v exceeds a certain threshold that depends on b and n but is relatively small). That is, decreasing the number of contributors and/or increasing their total share of the reward results in increasing group effort. Moreover, analytical derivation and numerical simulations strongly suggest that the derivative of v crit with respect to X is positive, so that the threshold valuation increases with decreasing the number of contributors. This leads to a recursive procedure for finding the equilibrium: (i) set for all ranks for which inequality (20) is not satisfied; (ii) using appropriate values of n e and v , find X * from equation (22); (iii) if there are ranks for which inequality (24) is not satisfied, set their contributions to zero, recompute n e and v , and return to step (ii). Assume there is only one contributor per group, say, individual of rank 1 so that n e =1 and . By evaluating the left-hand side of equation (22) at , one can show that the resulting expression is positive and thus the corresponding root of equation (22), that is, , is larger than bnv 1 . In this case, the contributor's fertility , while for all other group members f j ≥1. This means that the share of reproduction of the dominant individual is smaller than 1/ n . As another illustration, assume that there are only two individuals per group ( n =2), which is a common set-up in reproductive skew theory [39] , [40] . Then, individual i contributes a positive effort only if its valuation If both individuals contribute, their joint and individual efforts are given by equations (18) and (19) with n =2. If only individual i contributes, its effort can be found from equation (22) with n =2, n e =1, v = v i and X = x i . Figure 1 illustrates the dependence of individual contributions x i and the shares of reproduction f i /( f 1 + f 2 ) on valuation. Numerical results We have not been able to get analytical results for models that would include both between-individual heterogeneity (in costs or valuations) and genetic relatedness. Instead, we studied the effects of these factors numerically. To produce the next generation, first we identified a ‘parental group’ for each ancestral group (by random and independent sampling with probabilities P j ). Then, for each female in the parental group, we identified two fathers for her two children (by random and independent sampling with probabilities ). To produce each offspring, free recombination was followed by mutation with a small probability. Mutational effects at each locus were drawn randomly and independently from a truncated normal distribution with zero mean. In numerical studies of the basic model, we used all possible combinations of the following parameter values: expected benefit per individual b =0.25, 0.5, 1.0; cost coefficient c =0.25, 0.5, 1.0; group size n =4, 8, 12; inequality parameter δ =0.25, 0.5, 1.0, 2.0, 4.0. We performed 10 runs for each parameter combination. Some parameters did not change: number of groups G =1,000, mutation rate μ =0.001 per gene per generation, standard deviation of the mutational effect σ μ =0.1. In models with hierarchical groups, all n genes controlling the efforts at different ranks were unlinked. The initial individual efforts were chosen randomly and independently from a uniform distribution on [0,0.05]. Simulations ran for 200,000 generations. To avoid the appearance of negative fitness values in numerical simulations, we introduced upper boundaries on individual efforts x i ,max =(1+ bnv i )/ c . We used a zero lower boundary on x i . Supplementary Figs 1–6 summarize the results for three different sets of simulations: (i) the basic model as outlined above ( Supplementary Figs 1 and 2 ), (ii) the model with decisiveness coefficient β =2 ( Supplementary Figs 3 and 4 ) and (iii) the model of an egalitarian population with the cost coefficients c i increasing linearly with rank ( Supplementary Figs 5 and 6 ). Within each set, we show separately the results for the case of no genetic relatedness ( Supplementary Figs 1, 3 and 5 ) and for the case of genetic relatedness resulting from male philopatry ( Supplementary Figs 2, 4 and 6 ). No genetic relatedness was obtained by enforcing random dispersal of male offspring in addition to random dispersal of female offspring. How to cite this article: Gavrilets, S. & Fortunato, L. A solution to the collective action problem in between-group conflict with within-group inequality. Nat. Commun. 5:3526 doi: 10.1038/ncomms4526 (2014).